Competition between heavy fermion and Kondo interaction in isoelectronic A-site-ordered perovskites With current research efforts shifting towards the 4 d and 5 d transition metal oxides, understanding the evolution of the electronic and magnetic structure as one moves away from 3 d materials is of critical importance. Here we perform X-ray spectroscopy and electronic structure calculations on A -site-ordered perovskites with Cu in the A -site and the B -sites descending along the ninth group of the periodic table to elucidate the emerging properties as d -orbitals change from partially filled 3 d to 4 d to 5 d . The results show that when descending from Co to Ir, the charge transfers from the cuprate-like Zhang-Rice state on Cu to the t 2g orbital of the B site. As the Cu d -orbital occupation approaches the Cu 2+ limit, a mixed valence state in CaCu 3 Rh 4 O 12 and heavy fermion state in CaCu 3 Ir 4 O 12 are obtained. The investigated d -electron compounds are mapped onto the Doniach phase diagram of the competing RKKY and Kondo interactions developed for the f -electron systems. Transition metal (TM) oxides host a diversity of fascinating phenomena [1] , [2] , [3] , [4] , [5] , [6] . Several possible formal oxidation states of the TM ions coupled with the innate ability to stabilize those states by structural network of oxygens give rise to a striking change in the TM–O orbital hybridization W , electron–electron correlations U and the charge transfer energy Δ [7] ; the subtle competition between W , U and Δ across the 3 d group of the periodic table is then responsible for a vast landscape of interesting magnetic and electronic ground states [1] , [4] , [8] . In traversing the periodic table within groups of the 3 d →4 d →5 d TM blocks, the additional degree of freedom, the spin–orbit (SO) interaction, λ gets activated and is predicted to foster a multitude of exotic electronic and topological phases of correlated matter [9] , [10] , [11] , [12] , [13] , [14] , [15] . Although the vast majority of these compounds contain TM ions at the B -site of the AB O 3 perovskite structure, it is now possible to synthesize a new family of compounds with formula unit , Fig. 1a , where the perovskite A -site is partially occupied by a TM ion, labelled A ′. Among this class of materials, ( A Cu 3 ) B 4 O 12 with Cu in the A ′ site have garnered considerable attention because of the presence of CuO 4 planes. Structurally, this family of compounds consists of two different magnetically active sublattices of TM ions: B O 6 octahedral units (forming a three-dimensional octahedral network as in the typical AB O 3 perovskite lattice) and the planar CuO 4 units coupled with B O 6 units via an apical oxygen (see Fig. 1a ). Depending on the choice of B -site ion, the materials exhibit exciting properties including giant dielectric constant ( B =Ti), exotic ferromagnetism ( B =Ge, Sn, Fe), valence fluctuation ( B =V), Mott physics ( B =Ru) and inter-site charge order ( B =Fe) to name a few [16] , [17] , [18] , [19] , [20] , [21] , [22] . They are also of particular interest owing to the preservation of the cubic lattice symmetry , despite large variations of the B -site ion including utilizing different TM series (3 d or 4 d or 5 d ) of the periodic table [23] . This provides a unique platform to investigate the emergence of the electronic and magnetic states; for example, in recent work on (CaCu 3 ) B 4 O 12 ( B =Cr, Co), it has been demonstrated that the Zhang-Rice quantum state (essential for hole doped high- T c superconductivity) can be realized in these compounds, despite the lack of the superconducting ground state [24] , [25] , [26] . 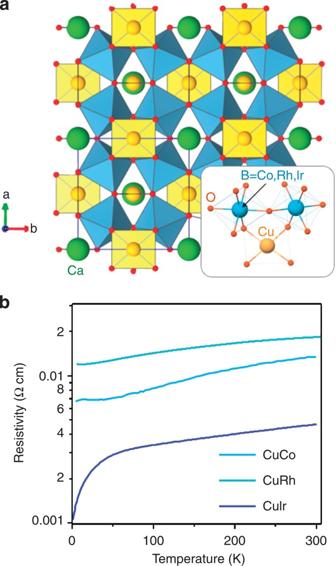Figure 1: Structure and properties of A-site-ordered perovskites. (a) Crystal structure ofA-site-ordered perovskites. Connection between CuO4planes and IrO6octahedra shown in the bottom right corner. (b) Temperature-dependent transport data for theB=Co, Rh, Ir samples displaying the anomalous behaviour for CCCIrO. CCCoO data taken from ref.22. CCIrO data taken from ref.27. Figure 1: Structure and properties of A-site-ordered perovskites. ( a ) Crystal structure of A -site-ordered perovskites. Connection between CuO 4 planes and IrO 6 octahedra shown in the bottom right corner. ( b ) Temperature-dependent transport data for the B =Co, Rh, Ir samples displaying the anomalous behaviour for CCCIrO. CCCoO data taken from ref. 22 . CCIrO data taken from ref. 27 . Full size image Very recently, Cheng et al. showed that this class of materials displays a crossover between the magnetic insulating and paramagnetic metallic states, depending on the Cu–O and B –O bond lengths [27] . It was further suggested that the CaCu 3 Ir 4 O 12 (CCIrO) compound, with the bond length within the crossover region, possesses anomalous electronic and magnetic properties arising presumably due to the interaction between the localized Cu and itinerant Ir states [23] . However, the mechanism by which the electronic structure transforms to create this emergent behaviour in CCIrO is not microscopically understood. In order to shed light on this interesting aspect, three isostructural and isoelectronic compounds whose B -site spans the ninth group of the periodic table, (CaCu 3 ) B 4 O 12 ( B =Co, Rh, Ir), were synthesized. Within the proposed phase diagram of Cheng et al. , B =Co occupies the paramagnetic metallic state, whereas CCIrO is at the crossover region as reflected for instance in anomalous d.c. transport properties shown in Fig. 1b (refs 22 , 27 ). In this paper, we investigate the electronic and magnetic structure of this new class of materials by a combination of resonant soft and hard X-ray absorption spectroscopy (XAS) on the Cu L-edge, O K-edge, and B -site L- and K-edges. Complementary first-principles calculations corroborate the experimental findings, providing microscopic understanding. Our results reveal that the unusual physical properties of these compounds are microscopically controlled by the degree of orbital occupancy and the strength of the B –O covalency. Spectroscopic results First, we discuss the evolution of the electronic structure of Cu. The Cu L 3 -edge XAS are presented in Fig. 2a (total fluorescence yield (TFY) available in supplementary Fig. 1 ). In accord with the previously reported results [24] for CaCu 3 Co 4 O 12 (CCCoO), the main absorption line at 931.4 eV arises due to absorption from the transition, where stands for a ligand hole whereas indicates a hole in the Cu 2 p core states. The low-energy shoulder around 930 eV arises from the transition; the d 9 transition accounting for 10% of the total peak area, indicating that there is a large Cu–O hybridization present in CCCoO. The line shape of the Cu L 3 absorption edge for CaCu 3 Rh 4 O 12 (CCRhO), containing the 4 d element Rh at the B -site, also contains a lesser and yet still significant contribution, giving a Cu valence of ~2.6+. The transport behaviour for this compound is quite similar to CCCO and points to CCRhO also being paramagnetic metallic ( Fig. 1b ). On the other hand, for CCIrO, the state is no longer present and the L 3 line shape is almost analogous to that recorded from purely ionic d 9 Cu 2+ charge state, agreeing with an earlier report utilizing electron energy loss spectroscopy [2] , [3] , [23] , [28] , [29] , [30] . This implies that the hole is no longer interacting with the final state, showing a significant reduction of the hole contribution to the hybridized orbital between Cu and O. Furthermore, the small multiplet split peak seen around ~940 eV for all Cu L 3 -edge spectra is due to a transition from the metastable 3 d 8 (Cu 3+ ) to the state; the small decrease in this 3 d 8 peak spectral weight in going from Co to Ir also indicates movement towards the ionic 3 d 9 state of Cu [29] , [30] , [31] . Taken as a whole, the Cu L 3 -edge data directly illustrate that in the presence of 4 d or 5 d orbitals, it is energetically more favourable to transfer the hole on to the B -site instead of stabilizing the Cu 3+ state, suggesting a strong change in covalency, as tabulated in Table 1 . 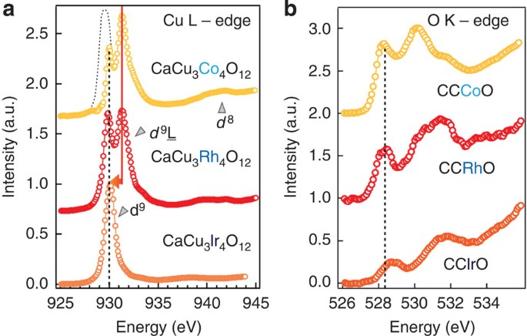Figure 2: Changing Cu and O valency as a function ofB-site. (a) Soft XAS on the Cu L-edge for all samples showing the changing Cu valence. The dotted line is the spectrum before the subtraction of the impurity peak (note that CCCoO TFY data and explanation of impurity peak originally given in ref.24). The dashed line indicates the energy of thed9peak. (b) XAS on the O K-edge showing both the reduction of the pre-peak on O and the shifting of the O 2p–Cu 3dand O 2p–B-sitedhybridized orbitals. The dashed line here indicates the energy of the O pre-peak associated with a doped hole. Figure 2: Changing Cu and O valency as a function of B -site. ( a ) Soft XAS on the Cu L-edge for all samples showing the changing Cu valence. The dotted line is the spectrum before the subtraction of the impurity peak (note that CCCoO TFY data and explanation of impurity peak originally given in ref. 24 ). The dashed line indicates the energy of the d 9 peak. ( b ) XAS on the O K-edge showing both the reduction of the pre-peak on O and the shifting of the O 2 p –Cu 3 d and O 2 p – B -site d hybridized orbitals. The dashed line here indicates the energy of the O pre-peak associated with a doped hole. Full size image Table 1 Experimental and theoretical values for the valence of Cu and the B -site for each compound. Full size table In the past, the electronic structure of Cu has been extensively studied in the context of high- T c superconducting cuprates, where it was also found that the reduction of ligand hole weight on Cu causes a decrease of the pre-peak intensity around 528 eV in the O K-edge XAS spectrum [32] , [33] , [34] , [35] . To track the movement of the hole in the present series of samples, we obtained O K-edge XAS spectra shown in Fig. 2b , with the post-edge normalized to 1 (at 540 eV). As immediately seen, the decrease of the relative intensity of the pre-peak indeed scales with the reduction of the ligand hole on Cu, implying a marked change in both bandwidth, W , and the charge transfer gap, Δ. The decrease of the pre-peak intensity can be rationalized in terms of a decreasing availability of empty states as the hole concentration on O decreases in moving from Co to Rh to Ir. Although the high-energy shoulder on the Cu L 3 peak disappears entirely for CCIrO, the oxygen pre-peak does not, which indicates the hybridization between the B -site and O is also significant, as Cu 2+ will not contribute to the pre-peak. The results of the O K-edge spectroscopy are thus in excellent agreement with the Cu L-edge observations. Another interesting observation is that the energy separation between the pre-peak and the peak around 530 eV increases from Co to Ir. The shift towards higher energy will be discussed in detail in the theory section and is attributed to the gradually increasing separation of the B -site bands (CCCoO) and both the B -site and Cu bands (CCRhO and CCIrO) from the O 2 p band. The movement of the hole away from Cu naturally implies a change in valency of the B -site ion. To verify this proposition and to corroborate the previous findings, we performed XAS on the L- and K-edges of Ir and Rh, respectively (Co was measured previously and found to be in the ~ 3.25+ state, after subtraction of an impurity peak [24] ). Moving to the 4 d compound, Rh K-edge XAS spectra have been simultaneously collected from the CCRhO sample and a standard SrRhO 3 reference sample. Although the line shape from CCRhO shares similarities with SrRhO 3 (Rh 4+ ), the difference in energy at 80% of the normalized absorption was found to be ~0.68 eV lower relative to SrRhO 3 , Fig. 3a (ref. 36 ). Based on this shift, and the shift of ~1.9 eV between Rh 3+ and Rh 4+ (see Supplementary Fig. 2 ), we conclude that the Rh valence state is indeed strongly mixed between 3+ and 4+, with a value of 3.64+ (±0.1). In conjunction with the Cu and O soft XAS, the entire Rh data set strongly supports the notion that the hole still largely resides on the O anion, but spreads to the hybridized orbital with Rh. Finally, the Ir L 3 edge (2 p 3/2 →5 d transition) recorded from CCIrO and SrIr(4+)O 3 is shown in Fig. 3b . As seen, the remarkably similar line shape and the energy peak position both confirm that Ir is in the 4+ state. The L 3 to L 2 branching ratio was found to be 3.79 (analysis shown in Supplementary Fig. 2 ) [9] , [11] . This value is similar to that found in several other iridate compounds and signifies a large SO coupling (SOC) as expected for a 5 d compound [9] , [11] , [37] , [38] . Overall, the Ir L-edge data are in excellent agreement with the Cu L-edge data stating the d 9 Cu 2+ ground state, with a much smaller d 8 contribution compared with the Rh and Co compounds; thus, in the CCIrO compound, the hole is now almost entirely transferred from the Cu 3 d –O 2 p state to the Ir 5 d –O 2 p hybridized orbital. The obtained valences for the B -sites are also listed in Table 1 . 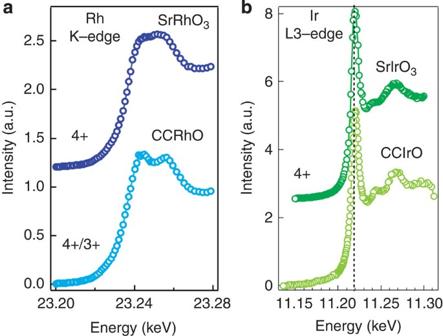Figure 3: Changing valency of theB-sites by hard XAS. (a) Hard XAS Rh K-edge measurements on the CCRhO and SrRhO3(4+) standard. (b) XAS on the Ir L3-edge for both CCIrO and a SrIrO3standard evidencing the nearly identical line shape and position indicating the 4+ valency. The dashed line shows the excellent agreement of the peak positions. Figure 3: Changing valency of the B -sites by hard XAS. ( a ) Hard XAS Rh K-edge measurements on the CCRhO and SrRhO 3 (4+) standard. ( b ) XAS on the Ir L 3 -edge for both CCIrO and a SrIrO 3 standard evidencing the nearly identical line shape and position indicating the 4+ valency. The dashed line shows the excellent agreement of the peak positions. Full size image Density functional theory (DFT) results Calculating the spin-polarized electronic structure of the three compounds, as a common feature, we find that the Cu d , B d and O p states are admixed, although the degree of admixture varies between the three compounds. Site-projected partial density of states is shown in Supplementary Fig. 3 (ref. 39 ). A direct inspection of the plot for CCCoO reveals that the states, which are strongly admixed with states, are empty in both spin-up and spin-down channels, thus lending strong support for the valence in CCCoO. This yields a mixed valence of 3.25+ on Co and the intermediate spin state with a magnetic moment of ~1.68 μ B . Moving towards the CCRhO compound, the admixture between the state and Rh states becomes markedly reduced compared with that of CCCoO. In this compound, the calculated Cu valence is found to be mixed between 2+ and 3+ (~2.5+), with Rh valence close to 3.6+. Unlike Co, magnetically Rh is found to be in the low spin state with a spin moment of 0.21 μ B and largely quenched orbital moment of 0.05 μ B . Finally, we consider the CCIrO. In sharp contrast to both Co and Rh, the mixing of the p states and the Ir d states is drastically reduced. This results in an almost pure p state occupied in one spin channel and empty in another, implying a Cu 2+ valence and nominal Ir 4+ valence. The spin moments at Ir and Cu sites are found to be 0.45 μ B and 0.65 μ B , respectively, with a rather large spin moment of 0.12 μ B on O, arising from strong hybridization with Ir. We note that ionic Ir 4+ is in the 5 d 5 configuration and has extensively been discussed in view of the interplay of strong SOC and correlation physics [9] , [10] , [11] , [12] , [13] , [14] , [15] . The large branching ratio of close to 3.8 signifies the presence of a large SOC at the Ir site, which is found to be common among many of the compounds of Ir 4+ in an octahedral environment, even when the compound is metallic as in IrO 2 (ref. 38 ). The orbital moment at the Ir site, calculated within the generalized gradient approximation (GGA)+U+SO, turned out to be 0.12 μ B , smaller than the spin moment with m orbital / m spin being 0.27. This is curious when compared with the values obtained in cases like BaIrO 3 (ref. 11 ). The structure and coupling mechanisms are, however, rather different between compounds like Sr 2 IrO 4 or BaIrO 3 and the present one. In the former examples, magnetic interactions are one- or two-dimensional Ir–Ir, whereas here they are Cu–Ir with three-dimensional connectivity. The dominance of hybridization produces an additional induced spin moment at the Ir site because of the presence of the magnetic ion Cu, a behaviour qualitatively similar to the case of La 2 CoIrO 6 , discussed in recent literature [37] . The presence of a significant SO interaction is found to mix up and down spins and destroys half-metallicity in CCIrO. We note here that inclusion of SOC allows for the non-collinear arrangement of spins. We have therefore carried out spin-polarized calculations assuming collinear as well as non-collinear spin arrangements. The calculated magnetic moments at various atomic sites, obtained in non-collinear calculations, turn out to be very similar to that obtained assuming simple collinear arrangement of spins. The spin magnetic moments are found to be similar to that obtained from collinear calculations within 1–2%, whereas the orbital magnetic moments are found to differ from that in collinear calculation by a maximum of 0.5%, providing confidence in the general conclusion drawn from the electronic structure calculations on the various valence and spin states, irrespective of the assumed spin arrangements. The evolution of the nominal valence of Cu from predominant 3+ ( d 9 L ) to 2+, as one moves from 3 d (Co) to 4 d (Rh) to 5 d (Ir) elements at the B -site, is controlled by mixing between B -site d states and p states and can be vividly visualized in the effective Wannier function plots shown in Fig. 4a (upper panel). As clearly seen, the Wannier functions centred at the Cu site have the orbital character of symmetry, and the tail is shaped according to the symmetry of the orbitals mixed with it. Specifically, moving from CCCoO to CCRhO to CCIrO, we find the weight at the tails centred at the B -site (marked by a circle) progressively diminishes. 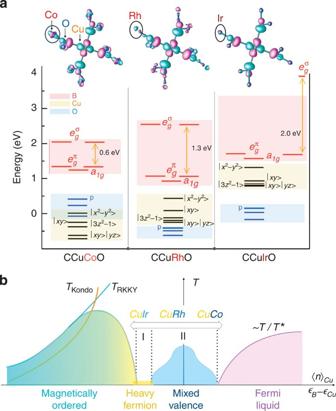Figure 4: Theoretical calculations and Doniach phase diagram. (a) Top panels: plots of effective Wannier functions for Op,orbitals for CCCoO, CCRhO and CCIrO. Plotted are the constant value surfaces with lobes of different signs coloured as cyan and magenta. The Cu,B- and O-sites are shown as green, red and blue coloued balls. Bottom panels: energy level positions of Cu d,B dand Opstates for CCCoO, CCRhO and CCIrO. (b) Doniach phase diagram showing the dependency on the Cu occupation. Figure 4: Theoretical calculations and Doniach phase diagram. ( a ) Top panels: plots of effective Wannier functions for O p , orbitals for CCCoO, CCRhO and CCIrO. Plotted are the constant value surfaces with lobes of different signs coloured as cyan and magenta. The Cu, B - and O-sites are shown as green, red and blue coloued balls. Bottom panels: energy level positions of Cu d, B d and O p states for CCCoO, CCRhO and CCIrO. ( b ) Doniach phase diagram showing the dependency on the Cu occupation. Full size image Microscopically, the nature of this peculiar unmixing/dehybridization effect between Cu–O and B -site in moving from 3 d to 4 d to 5 d element at the B -site can be further elucidated by considering the energy level positions of B d , Cu d and O p states (see Fig. 4a (bottom panel)). As mentioned above, the octahedral crystal field coupled with the trigonal distortion separates the B d states into doubly degenerate , and singly degenerate a 1 g ones, whereas the square planar geometry of the CuO 2 plane breaks the Cu d states into and the rest, with being of the highest energy. In progressing from CCCoO to CCRhO to CCIrO, the relative position of with respect to O p states increases, driven by the pushing down of O p states because of the increased crystal field splitting ( splitting) at the B -site. This, in turn, makes the hybridization between the Cu sublattice and B sublattice weaker and weaker as those ions communicate via the intervening oxygen. This highlights a key difference between CCIrO and CaCu 3 Ru 4 O 12 , where for the latter it was found that the suspected Kondo-like physics was unlikely due to a strong mixing of Cu with O [40] , [41] . Similar to that of high- T c cuprates, for CCCoO, the O p states are positioned above , placing Cu in to a negative charge transfer regime, which promotes a high- T c cuprate-like state akin to the Zhang-Rice singlet state [24] , [25] , [26] , [42] . The progressive weakening of covalency between the B sublattice and Cu–O sublattice, as one moves from CCCoO to CCRhO to CCIrO, makes the spread of the effective Wannier function (top panel of Fig. 4a ) in the case of Ir dramatically reduced compared with either Co or Rh. Unified picture Finally, the element-resolved spectroscopic results combined with the ab-initio calculations prompts us to build a unified framework to explain their emergent physical behaviour. Although an earlier study utilizing electron energy loss spectroscopy found small changes between 3–4–5 d A-site-ordered perovskites from different columns [23] , our study reveals that upon ascending a column of the periodic table from Ir to Co, the orbital occupation changes from practically ionic for CCIrO to the non-magnetic cuprate Zhang-Rice-like state with for CCCoO, as supported by experimentally and theoretically deduced valences listed in Table 1 . Along with it, these localized and magnetically active Cu d states in CCIrO shift towards the Fermi surface demonstrating a rapid change in hybridization compared with both CCRhO and CCCoO. On the opposite end, such a drastic change in the Cu orbital occupation results in the mixed valence intermediate spin state of Co 3.25+ , mixed valence Rh~3.7+ but ionic Ir 4+ (5 d 5 ). These findings allow us to place the three compounds under discussion in the context of the Doniach phase diagram depicted in Fig. 4b , where the fundamental control parameter is the average occupation ‹ n › Cu of the orbital modulated by the hybridization from the strongly mixed B -site d - and O p -bands [43] , [44] , [45] . In the modern version of the Doniach phase diagram, interesting physics involving heavy fermions manifests itself as a competition between the Kondo liquid and spin liquid behaviour mediated by chemical doping, whereas very little attention has been given to the mixed valency regime, particularly in d -electron systems and in the absence of doping [43] , [44] , [45] , [46] , [47] , [48] . In this framework, the overall ground state is defined by the competition between RKKY-type magnetic exchange between magnetic holes on Cu with the Kondo screening by conduction carries from the B –O sublattices. For CCIrO, with a S =1/2 d -hole localized on Cu, the large magnetic exchange is comparable in strength with the Kondo screening, resulting in the strongly enhanced effective mass observed with transport and thermal measurements [27] . Thus, Cheng et al. firmly placed CCIrO into the heavy fermion regime I in Fig. 4b with the antiferromagnetic local moment short-range magnetism [23] , [27] . In moving from Ir to Rh and Co, the Kondo energy scale begins to gain because of the collective hybridization of Cu d-holes into the ZR singlets. With the strong reduction in the orbital occupation, both CCRhO and CCCoO enter the regime II of mixed valency (or Kondo liquid phase) in Fig. 4b . Unlike regime I, in the mixed valence regime quantum fluctuations between different electronic configurations are highly relevant; in this regime, the local electronic and magnetic structure of Kondo centres (Cu) is defined by the redistribution of electrons between Cu d states and electrons from the strongly hybridized d- and p -states of Rh (Co) and O, that is, |3 d 9 , S =1/2› versus . The conjectured microscopic framework that links the electronic and magnetic ground state of the A -site perovskites with macroscopic behaviour opens a path in designing emergent-ordered phases with heavy fermion behaviour, quantum criticality and unconventional superconductivity in the magnetic Kondo lattice of cuprate-like moments. To summarize, we performed XAS measurements and first-principles calculations on a series of A -site-ordered perovskites, chemical formula CaCu 3 B 4 O 12 , spanning one period of the periodic table. Surprisingly, we find that the materials fit well within the Doniach phase diagram, being controlled by the hole count on Cu, leading to the conclusion that the competition between RKKY and Kondo effects is responsible for the anomalous behaviour observed in the CCIrO compound. Sample preparation All samples used in the present study were prepared under high-pressure and high-temperature conditions with a Walker-type multianvil module (Rockland Research Co.). The A-site-ordered perovskites CCCoO, CCRhO and CCIrO were obtained under P =9 GPa and T =1,000–1,300 °C; the reference perovskites SrRhO 3 and SrIrO 3 were obtained at 8 GPa, 1,200 °C and 6 GPa, 1,000 °C, respectively. About 30 wt.% KClO 4 acting as oxidizing agent were added for synthesizing the compounds containing Co and Rh. The resultant KCl was washed away with deionized water. Phase purity of the above samples was examined with powder X-ray diffraction at room temperature with a Philips Xpert diffractometer (Cu K α radiation). All the A-site-ordered perovskites adopt a cubic structure with lattice parameter increasing progressively from a =7.1259(3) Å for M =Co to a =7.3933(1) Å for M =Rh, and to a =7.4738(1) Å for M =Ir. On the other hand, the reference perovskites crystallize into the orthorhombic Pbnm structure with unit-cell parameters a =5.5673(1) Å, b =5.5399(2) Å and c =7.8550(2) Å for SrRhO 3 , and a =5.5979(1) Å, b =5.5669(1) Å and c =7.8909(1) Å for SrIrO 3 , respectively. X-ray measurements XAS measurements were carried out on the polycrystalline samples in the soft X-ray branch at the 4-ID-C beamline in the bulk-sensitive TFY and total electron yield modes, with a 0.1 eV (0.3 eV) resolution at the O K-edge (Cu L-edge), at the Advanced Photon Source in Argonne National Laboratory. Measurements were taken on the Cu L-edge and O K-edge for all samples, and all measurements shown here were obtained in total electron yield mode (TFY available in Supplementary Fig. 1 ). To measure the 4 d and 5 d B -site valences, hard XAS measurements with a 1.5(3) eV resolution were taken at the 4-ID-D beamline in transmission (fluorescence) mode for Ir (Rh). Computational details In the first-principles DFT calculations, we have primarily used the plane wave basis set and pseudo-potentials as implemented in the Vienna Ab-initio Simulation Package [49] . The exchange-correlation function was chosen to be that of the GGA implemented following the parametrization of Perdew-Burke-Ernzerhof [50] . The electron–electron correlation beyond GGA was taken into account through improved treatment of GGA+ U calculation within the + U implementation of Dudarev et al. [51] For the plane wave-based calculations, we used projector augmented wave [52] potentials. The wave functions were expanded in the plane wave basis with a kinetic energy cutoff of 600 eV and Brillouin zone (BZ) summations were carried out with a 6 × 6 × 6 k-mesh. A U -value of 5 eV on Cu site was used. For the U -value on the B site, a value of 4 eV was used for the 3d element Co and 1–2 eV was used for 4 d and 5 d elements, Rh and Ir. The obtained results were verified in terms of variation of U parameter. The Hund’s rule coupling J was fixed to 0.8 eV. The plane wave results were verified in terms of full-potential linearized augmented plane wave method as implemented [53] in WIEN2k. For FLAPW calculations, we chose the augmented plane wave+lo as the basis set and the expansion in spherical harmonics for the radial wave functions was taken up to l =10. The charge densities and potentials were represented by spherical harmonics up to l =6. For BZ integration, we considered about 200 k-points in the irreducible BZ and modified tetrahedron method was applied [54] . The commonly used criterion for the convergence of basis sets relating the plane wave cutoff, K max , and the smallest atomic sphere radius, R MT , R MT * K max , was chosen to be 7.0. Spin–orbit coupling has been included in the calculations in scalar relativistic form as a perturbation to the original Hamiltonian. To estimate the positions of the Cu d , B d and O p energy levels as well as the plots of the effective Wannier functions for B d states, we used muffin-tin orbital (MTO)-based N-th order MTO (NMTO) [55] -downfolding calculations. Starting from full DFT calculations, NMTO-downfolding arrives at a few-orbital Hamiltonian by integrating out degrees, which are not of interest. It does so by defining energy-selected, effective orbitals, which serve as Wannier-like orbitals defining the few-orbital Hamiltonian in the downfolded representation. NMTO technique, which is not yet available in its self-consistent form, relies on the self-consistent potential parameters obtained out of linear MTO [56] calculations. The results were cross-checked among the calculations in three different basis sets in terms of total energy differences, density of states and band structures. How to cite this article: Meyers, D. et al. Competition between heavy fermion and Kondo interaction in isoelectronic A-site-ordered perovskites. Nat. Commun. 5:5818 doi: 10.1038/ncomms6818 (2014).